CD95 and CD95L promote and protect cancer stem cells CD95 (APO-1/Fas) is a death receptor used by immune cells to kill cancer cells through induction of apoptosis. However, the elimination of CD95 or its ligand, CD95L, from cancer cells results in death induced by CD95R/L elimination (DICE), a type of cell death that resembles a necrotic form of mitotic catastrophe suggesting that CD95 protects cancer cells from cell death. We now report that stimulation of CD95 on cancer cells or reducing miR-200c levels increases the number of cancer stem cells (CSCs), which are more sensitive to induction of DICE than non-CSC, while becoming less sensitive to CD95-mediated apoptosis. In contrast, induction of DICE or overexpression of miR-200c reduces the number of CSCs. We demonstrate that CSCs and non-CSCs have differential sensitivities to CD95-mediated apoptosis and DICE, and that killing of cancer cells can be maximized by concomitant induction of both cell death mechanisms. CD95 (Fas/APO-1) is a death receptor that induces apoptosis mainly in immune cells through a well-characterized pathway [1] , [2] , which involves the formation of a death-induced signalling complex upon binding with its ligand, CD95L [2] , [3] . In addition, immune cells can kill cancer cells by using CD95L [4] . However, CD95 is also emerging as a tumour promoter that enhances growth, motility and invasion of cancer cells by activating various non-apoptotic signalling pathways including NF-κB, mitogen-activated protein kinases and Src-family kinases [5] , [6] , [7] . Furthermore, CD95 engagement was reported to accelerate normal liver regeneration following partial hepatectomy [8] , [9] . Additional evidence of a pro-survival function of CD95 and CD95L signalling in normal cells came from the analysis of stem cells (SCs). It was found that induction of CD95 signalling in neuronal SC did not cause death but rather increased the survival of SC, while, conversely, deletion of CD95 resulted in reduced neurogenesis [10] . Finally, CD95/TNFRSF6 was identified as a candidate marker in a serial analysis of gene expression profiling of human embryonic SC, which included well-established SC markers such as LIN28, OCT4, NANOG and SOX2 (ref. 11 ). We previously reported that CD95 contributes to tumour growth in vitro and in vivo in genetic mouse models of ovarian and liver cancer [9] . We have subsequently demonstrated that when either CD95 or CD95L are eliminated cancer cells die through a process we have coined DICE (for death induced by CD95R/L elimination) [12] . DICE is a necrotic form of mitotic catastrophe characterized by cell swelling and reactive oxygen species production followed by DNA damage, activation of caspase-2 and loss of mitochondrial outer membrane potential [12] . DICE appears to be a fundamental mechanism, since it was consistently detected in all cancer cells investigated and in an in vivo mouse model of low-grade ovarian cancer. More recently, we proposed that DICE is part of a cancer surveillance mechanism that ensures that cells undergoing neoplastic transformation never lose CD95, which would prevent CD95L-expressing immune cells from eliminating such cells [13] . In light of the above-mentioned role of CD95 in SCs, and based on the link between CD95 signalling and the differentiation stage of cancer [14] , we asked whether DICE may differentially affect cancer cells depending on their differentiation status, that is, cancer stem cells (CSCs) versus more differentiated or normal cancer cells (non-CSCs). We now report that stimulation of CD95 on multiple kinds of tumour cells induces a conversion from non-CSCs to CSCs with a concomitant reduction in sensitivity to CD95-mediated apoptosis and increased susceptibility to DICE. Induction of DICE in both cell lines and primary cancer cells resulted in a depletion of CSCs. In breast cancer, we could connect this novel function of CD95/CD95L to the activity of miR-200, a micro(mi)RNA previously linked to both epithelial-to-mesenchymal transition (EMT) and CSCs [15] , [16] , [17] . Our data suggest that the two death mechanisms, DICE and CD95-mediated apoptosis, have opposing roles in eliminating CSCs and non-CSCs. As a consequence, the induction of both DICE and CD95-mediated apoptosis kills cancer cells more effectively than either mechanism alone. CD95 stimulation increases the number of CSCs We previously reported that cancer cells die when either CD95 or CD95L is eliminated [12] . However, not all cells in a culture died, suggesting that subpopulations exist with differential sensitivity to DICE. Interestingly, two clones of the mouse colon cancer cell line CT26 expressing large quantities of human CD95L (CT26L, clones 18 and 22) died quantitatively after expression of the CD95L-specific shRNA L3 (ref. 12 ). We recently reported that stimulation of CD95 on cancer cells caused a reduction in the expression of the let-7 family of miRNAs, which maintains differentiation of cells and prevents generation of SCs [18] , [19] . We therefore wondered whether the constant stimulation of endogenous CD95 in CT26L cells by exogenous CD95L rendered the cells more sensitive to DICE by increasing their stemness. CSCs are known to be able to grow as tumour spheres when plated under low adherence conditions [20] . Interestingly, the two CT26L clones formed spheres more readily than parental CT26 cells without an increase in their proliferative capacity ( Fig. 1a,b ). On the basis of this observation we tested whether prolonged stimulation of cancer cells through CD95 produced an increase in the numbers of CSCs. We cultured three cancer cell lines representing breast (MCF-7), colon (HCT116) and renal (CAKI-1) cancer in the presence of the agonistic antibody anti-APO-1 or the highly active leucine zipper-tagged CD95L (LzCD95L), both of which can activate canonical apoptotic signalling through CD95. We expected this treatment to eliminate all CD95 apoptosis-sensitive cells after a few hours of treatment. In order to maintain a high concentration of the two anti-CD95 agonists, media was replaced every 3–4 days with fresh anti-APO-1 or LzCD95L ( Fig. 1c ). Consistent with the moderate-to-weak CD95 apoptosis sensitivity of the three cell lines [21] , after a 3-day incubation only a small number of dead cells could be detected. Surprisingly, although every time fresh anti-APO-1 or LzCD95L was added, and a substantial number of cells died, the overall cell numbers increased. One possible explanation for this phenomenon was that while the culture conditions constantly eliminated cells that were sensitive to CD95-mediated apoptosis, the surviving apoptosis-resistant cells differentiated and gave rise to apoptosis-sensitive as well as apoptosis-resistant cells. This would be consistent with a known property of stem-like cells: asymmetric division ( Fig. 1d , Supplementary Fig. 10 ). Evidence that this was indeed the case was obtained from western blot analysis. MCF-7 cells treated for 2 weeks with LzCD95L showed a significant increase in CD44 and a concomitant decrease in CD24 expression ( Fig. 1d ), compatible with the established phenotype (CD44 high CD24 low ) of breast CSCs [20] . An increase in CSCs in the CD95-stimulated cells was also consistent with the upregulation of CSC markers SOX2 (ref. 22 ) and ZEB1 (ref. 23 ; Fig. 1d ). An increase in CD44 high CD24 low cells was also detected in MCF-7 and T47D cells using flow cytometry after stimulation with anti-APO-1 for 2 weeks. Both CD95-stimulated MCF-7 and T47D cells showed an increased ability to form spheres under these conditions ( Fig. 1e,f ). 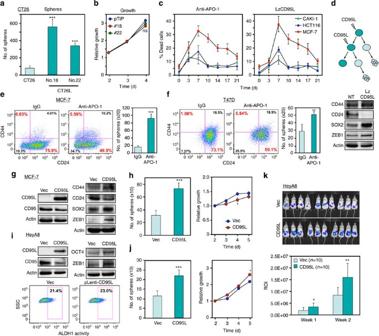Figure 1: Stimulation of CD95 increases the number of CSCs. (a) Quantification of spheres of CT26 cells and two CT26L clones after 1 week of culture. Histograms represent mean+s.d. of three independent cultures (two experiments). (b) Proliferation (MTS) assay in cells as inabut grown under adherence conditions (normalized to day 1). Data represent mean±s.d. of four independent cultures. (c) Cell death quantification (percent Trypan blue-positive cells) of different cells grown in the presence of anti-APO-1 or leucine zipper-tagged CD95L (LzCD95L) over 3 weeks. Data represent mean±s.d. of four independent cultures. (d)Top:proposed model to explain the effects of constant CD95 stimulation, inducing cell death in one population (light blue) and expansion in another.Bottom:western blot analysis of MCF-7 cells either untreated or treated for 2 weeks with LzCD95L. (e,f)Left:flow cytometry analysis of surface staining of MCF-7 (e) and T47D (f) cells for CD24 and CD44, 2 weeks after continuous treatment with IgG control or with anti-APO-1. Gates are based on isotype controls. Three independent experiments were analysed.Right:quantification of spheres obtained from cells cultured in suspension as inein sphere-forming media for 1 week. (g) Western blot analysis of MCF-7 cells infected with control or CD95L expression lentiviral vector. (h)Left:quantification of spheres of MCF-7-Vec or MCF-7-CD95L cells. Histograms represent mean+s.d. of three independent cultures (two experiments).Right:MTS proliferation assay. Histograms represent mean±s.d. of four independent cultures. (i)Top:western blot analysis of HeyA8-Vec or HeyA8-CD95L cells.Bottom:ALDH1 activity of the same cells. Gates are based on samples co-treated with DEAB-inactivating reagent. Two independent experiments were analysed. (j)Left:quantification of spheres of HeyA8-Vec or HeyA8-CD95L cells. Histograms represent mean+s.d. of three independent cultures (two experiments).Right:MTS proliferation assay. Histograms represent mean±s.d. of four independent cultures. (k) Quantification of the total luminescence in the regions of interests (ROIs) in mice injected with luciferase-expressing HeyA8-Vec or HeyA8-CD95L cells for the indicated time. The images show the mice 2 weeks after tumour injection. Histograms represent mean+s.d. (data from two experiments were pooled).Pvalues were calculated byt-test. *P<0.05; **P<0.001; ***P<0.0001. Figure 1: Stimulation of CD95 increases the number of CSCs. ( a ) Quantification of spheres of CT26 cells and two CT26L clones after 1 week of culture. Histograms represent mean+s.d. of three independent cultures (two experiments). ( b ) Proliferation (MTS) assay in cells as in a but grown under adherence conditions (normalized to day 1). Data represent mean±s.d. of four independent cultures. ( c ) Cell death quantification (percent Trypan blue-positive cells) of different cells grown in the presence of anti-APO-1 or leucine zipper-tagged CD95L (LzCD95L) over 3 weeks. Data represent mean±s.d. of four independent cultures. ( d ) Top: proposed model to explain the effects of constant CD95 stimulation, inducing cell death in one population (light blue) and expansion in another. Bottom: western blot analysis of MCF-7 cells either untreated or treated for 2 weeks with LzCD95L. ( e , f ) Left: flow cytometry analysis of surface staining of MCF-7 ( e ) and T47D ( f ) cells for CD24 and CD44, 2 weeks after continuous treatment with IgG control or with anti-APO-1. Gates are based on isotype controls. Three independent experiments were analysed. Right: quantification of spheres obtained from cells cultured in suspension as in e in sphere-forming media for 1 week. ( g ) Western blot analysis of MCF-7 cells infected with control or CD95L expression lentiviral vector. ( h ) Left: quantification of spheres of MCF-7-Vec or MCF-7-CD95L cells. Histograms represent mean+s.d. of three independent cultures (two experiments). Right: MTS proliferation assay. Histograms represent mean±s.d. of four independent cultures. ( i ) Top: western blot analysis of HeyA8-Vec or HeyA8-CD95L cells. Bottom: ALDH1 activity of the same cells. Gates are based on samples co-treated with DEAB-inactivating reagent. Two independent experiments were analysed. ( j ) Left: quantification of spheres of HeyA8-Vec or HeyA8-CD95L cells. Histograms represent mean+s.d. of three independent cultures (two experiments). Right: MTS proliferation assay. Histograms represent mean±s.d. of four independent cultures. ( k ) Quantification of the total luminescence in the regions of interests (ROIs) in mice injected with luciferase-expressing HeyA8-Vec or HeyA8-CD95L cells for the indicated time. The images show the mice 2 weeks after tumour injection. Histograms represent mean+s.d. (data from two experiments were pooled). P values were calculated by t -test. * P <0.05; ** P <0.001; *** P <0.0001. Full size image To test whether stable expression of CD95L would also increase the proportion of CSCs in cancer cells, MCF-7 cells were infected with a lentivirus coding for membrane-bound human CD95L. Western blot analysis of the surviving cells demonstrated efficient transduction with CD95L, resulting in a moderate downregulation of CD95 ( Fig. 1g , Supplementary Fig. 10 ), presumably because of the known internalization and degradation of CD95 upon continued stimulation by CD95L [24] . Analysis of the breast CSC markers CD44 and CD24, as well as SOX2 and ZEB1, indicated the emergence of the breast CSC phenotype in CD95L-overexpressing cells ( Fig. 1g , Supplementary Fig. 10 ). This phenotype was further confirmed by the upregulation of ALDH1-positive cells ( Supplementary Fig. 1a ). When MCF-7-CD95L and MCF-7-vec cells were subjected to a tumour sphere-forming assay, cells expressing exogenous CD95L formed significantly more spheres than cells infected with an empty vector, confirming that CD95-expressing cells had acquired increased CSC properties ( Fig. 1h ). Proliferation assays indicated that this phenotypic switch did not involve increased growth ( Fig. 1h ). Similar results were obtained when CD95L was overexpressed in the ovarian cancer cell line HeyA8. HeyA8-CD95L cells displayed increased expression of the CSC markers OCT4 and ZEB1 together with a moderate increase in aldehyde dehydrogenase (ALDH1) activity ( Fig. 1i , Supplementary Fig. 11 ). They also exhibited increased sphere formation ability in the absence of a significant impact on cell growth ( Fig. 1j ). As expected, both MCF-7- and HeyA8-overexpressing CD95L had increased resistance to CD95-mediated apoptosis when compared with vector-infected cells ( Supplementary Fig. 1b ). To test whether cells with a higher CSC content would also form tumours more readily in mice, we orthotopically injected nonobese diabetic (NOD)-gamma (NSG) mice with CD95L-expressing HeyA8 cells. This resulted in increased tumour growth 2 weeks after tumour cell injection ( Fig. 1k ). Thus, the evidence indicates that continued stimulation of CD95 over long periods of time increases the number of CSCs resulting in a gradual loss of cells that were sensitive to CD95-mediated apoptosis, in turn allowing accelerated growth of tumours in vivo . The emergence of CSCs in CD95-stimulated cancer cell populations could have three explanations: (1) CSCs are less sensitive to CD95-mediated apoptosis, and stimulating cells through CD95 eliminates CD95 apoptosis-sensitive cells, thereby enriching for CSCs; (2) CSC cells respond to CD95 stimulation with growth, resulting in their expansion; or (3) stimulation of CD95 on cancer cells induces their dedifferentiation resulting in the acquisition of CSC traits. To test whether the emergence of CSCs was because of a differential sensitivity of CSCs and non-CSCs to CD95-mediated apoptosis, MCF-7 cells were treated for 1 week with anti-APO-1 in the presence or absence of the oligospecific caspase inhibitor zVAD-fmk (zVAD). Although zVAD completely blocked canonical CD95-mediated apoptosis ( Supplementary Fig. 2a ), apoptosis inhibition did not prevent the increase in the percentage of CSCs ( Supplementary Fig. 2b ) pointing at an effect not completely dependent on differential sensitivity of CSCs and non-CSCs to CD95-mediated apoptosis. To test whether an increase in proliferation accounted for the emergence of CSCs, we labelled MCF-7 cells with carboxyfluorescein succinimidyl ester (CFSE), and stimulated the cells with anti-APO-1 ( Supplementary Fig. 2c ). This resulted in an increase in the numbers of a slow-proliferating (highly CFSE-retaining) population of CD44 high cells (from 5.8 to 16.5%). These data suggested that increased proliferation did not account for the emergence of CSCs following stimulation through CD95 and that CD95 stimulation caused dedifferentiation of non-CSCs. We cannot exclude at this point, however, that CD95 stimulation increased the ability of CSCs to asymmetrically divide. Stimulation through CD95 stabilizes CSCs It is now established, at least for breast cancer, that CSCs not only give rise to non-CSCs, but that non-CSCs can also supply cancer cell populations with CSCs through a spontaneous dedifferentiation process with features of EMT [25] , [26] . To test whether CD95 stimulation affects this process, we sought to isolate CSCs through their specific properties rather than by CSC markers or sphere-forming assays. Both techniques have recently come under scrutiny as they do not allow a full description of CSCs [27] , [28] , [29] , [30] , [31] . In the context of breast cancer, a specific miRNA, miR-200, is an established marker and functional regulator of both EMT and CSCs [15] , [17] , [32] . To isolate and track breast cancer cells through the expression of miR-200 family miRNAs, we developed a lentiviral miRNA sensor to monitor the expression and the activity of miR-200 in living cells. ZEB2 has been previously associated with CSCs [33] . We designed the sensor plasmid to express DsRed (red fluorescence) under the control of the fused ZEB2 3′-untranslated repeat (UTR) fragment containing three wild-type seed matches for miR-200b,c,429. As a nontargeting control, we fused green-fluorescent protein (GFP; green fluorescence) to the same 3′-UTR fragment with all three miR-200 seed matches inactivated by mutation at three positions (DsRed wt GFP mut ) ( Supplementary Fig. 3a ). When the DsRed wt GFP mut sensor plasmid was transfected into 293T cells, simultaneous transfection of pre-miR-200c suppressed DsRed protein with no effect on the expression of GFP, confirming specificity of the sensor ( Supplementary Fig. 3b,c ). The sensor detected subnanomolar changes in transfected pre-miR-200c ( Supplementary Fig. 3b ). We found that the miR-200 sensor system was able to equally detect the changes in the miR-200b, miR-200c and miR-429 subfamilies but did not respond to the expression of the miR-200a and miR-141 subfamilies ( Supplementary Fig. 4 ). We tested the ability of the sensor to detect endogenous levels of miR-200 by infecting MCF-7 cells with the lentiviral vector and by both the DsRed wt GFP mut and the DsRed mut GFP wt configurations to exclude positional effects of the fluorophores. The results indicated that both constructs were sensitive to miR-200 expression ( Supplementary Fig. 5a ). Using this sensor to analyse the ‘miR-200 high’ cells MCF-7 and the ‘miR-200 low’ cells HeyA8 ( Supplementary Fig. 5b ), the two cell lines showed very different repression of red fluorescence, establishing effective and reliable monitoring of miR-200 expression in an endogenous setting using the miRNA sensor ( Supplementary Fig. 5c ). Finally, to test whether the sensor could also detect dynamic changes in miR-200 expression at endogenous levels, we treated MCF-7 cells with a locked nucleic acid (LNA) oligonucleotide to inhibit miR-200 (ref. 15 ; Supplementary Fig. 5d ). This resulted in a significant increase in the red/green population in the LNA200-treated cells infected with the DsRed wt GFP mut plasmid ( Supplementary Fig. 5e,f ), confirming the specificity and sensitivity of the sensor. These data confirmed that the miRNA sensor was selective for miR-200 and that it detected changes in endogenous miR-200 expression levels. We sought to test whether the miRNA sensor could be used to track and isolate CSCs. Consistent with published reports [17] , CD44 high CD24 low cells from MCF-7 showed reduced miR-200 levels ( Fig. 2a ). When infected with the sensor, miR-200 high expressing non-CSCs were expected to be only green, whereas miR-200 low expressing CSCs should be red/green. We found that both red/green (miR-200 low) MCF-7 and T47D cells had a higher ability to form spheres than green-only (miR-200 high) cells, and they showed significant enrichment of CD44 high CD24 low cells, thus, confirming that CSCs can be enriched through the activity of miR-200 ( Fig. 2b ). It has been reported that spheres of MCF-7 cells show reduced miR-200 levels [34] . As a further confirmation, we grew MCF-7 cells infected with the DsRed wt GFP mut virus in mammospheres and analysed their fluorescence; we found that the expression of DsRed (otherwise suppressed in adherent cells) was highly increased ( Fig. 2c , compared with Fig. 2b ). We confirmed this result using MCF-7 cells expressing the sensor in the opposite configuration DsRed mut GFP wt ( Supplementary Fig. 5g ) excluding a positional effect of the fluorophores. 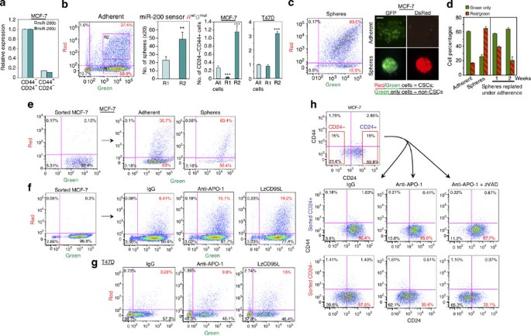Figure 2: CD95/CD95L regulates the plasticity of CSCs. (a) miR-200b and miR-200c expression levels in flow cytometry-sorted CD44lowCD24highand CD44highCD24lowMCF-7 cells, assessed with real-time PCR. Histograms represent mean+s.d. of three independent measurements. Two independent experiments were performed. (b)Left: flow cytometry quantification of green and red fluorescence of MCF-7 cells infected with the miR-200 DsRedwtGFPmutsensor. Gates are based on uninfected cells. Three independent experiments were performed.Centre: sphere quantification of cells in gates R1 and R2 flow cytometry-sorted and seeded for sphere formation for 1 week.Right: percent of CD44highCD24lowMCF-7 and T47D cells in the R1 and R2 gates. Histograms represent mean+s.d. of three independent cultures. (c) Red/green quantification (left) and representative images (right) of MCF-7 cells carrying the miR-200 DsRedwtGFPmutsensor grown for 7 days under adherence or sphere-forming conditions. Scale bar represents 100 μm. Gates are based on uninfected cells. Histograms represent mean+s.d. Two independent experiments were performed. (d)Left:percent of green-only and red/green cells in DsRedwtGFPmutMCF-7 cultures quantified under the indicated conditions.Right:red/green quantification of the MCF-7 spheres replated under adherence conditions for 1 or 2 weeks. Histograms represent mean+s.d. Two independent experiments were performed. (e) Red/green quantification of flow cytometry-sorted DsRedwtGFPmutMCF-7 green-only cells plated under adherence or sphere-forming conditions for 7 days. (f,g) Red/green quantification of flow cytometry-sorted green-only DsRedwtGFPmutMCF-7 cells (f) and T47D cells (g) grown for 10 days in the presence of IgG control, anti-APO-1 or LzCD95L. Gates are based on uninfected cells. Two independent experiments were performed. (h) Histograms of flow cytometry-sorted MCF-7 cells (for CD24 expression, as indicated) treated with IgG, anti-APO-1 and anti-APO-1+zVAD for 1 week and stained for CD24/CD44. Gates are based on isotype controls.Pvalues were calculated byt-test. **P<0.001; ***P<0.0001. Figure 2: CD95/CD95L regulates the plasticity of CSCs. ( a ) miR-200b and miR-200c expression levels in flow cytometry-sorted CD44 low CD24 high and CD44 high CD24 low MCF-7 cells, assessed with real-time PCR. Histograms represent mean+s.d. of three independent measurements. Two independent experiments were performed. ( b ) Left : flow cytometry quantification of green and red fluorescence of MCF-7 cells infected with the miR-200 DsRed wt GFP mut sensor. Gates are based on uninfected cells. Three independent experiments were performed. Centre : sphere quantification of cells in gates R1 and R2 flow cytometry-sorted and seeded for sphere formation for 1 week. Right : percent of CD44 high CD24 low MCF-7 and T47D cells in the R1 and R2 gates. Histograms represent mean+s.d. of three independent cultures. ( c ) Red/green quantification (left) and representative images (right) of MCF-7 cells carrying the miR-200 DsRed wt GFP mut sensor grown for 7 days under adherence or sphere-forming conditions. Scale bar represents 100 μm. Gates are based on uninfected cells. Histograms represent mean+s.d. Two independent experiments were performed. ( d ) Left: percent of green-only and red/green cells in DsRed wt GFP mut MCF-7 cultures quantified under the indicated conditions. Right: red/green quantification of the MCF-7 spheres replated under adherence conditions for 1 or 2 weeks. Histograms represent mean+s.d. Two independent experiments were performed. ( e ) Red/green quantification of flow cytometry-sorted DsRed wt GFP mut MCF-7 green-only cells plated under adherence or sphere-forming conditions for 7 days. ( f , g ) Red/green quantification of flow cytometry-sorted green-only DsRed wt GFP mut MCF-7 cells ( f ) and T47D cells ( g ) grown for 10 days in the presence of IgG control, anti-APO-1 or LzCD95L. Gates are based on uninfected cells. Two independent experiments were performed. ( h ) Histograms of flow cytometry-sorted MCF-7 cells (for CD24 expression, as indicated) treated with IgG, anti-APO-1 and anti-APO-1+zVAD for 1 week and stained for CD24/CD44. Gates are based on isotype controls. P values were calculated by t -test. ** P <0.001; *** P <0.0001. Full size image As expected, CSC (green/red) cells isolated by culturing MCF-7 cells under sphere-forming conditions reverted to green-only cells when returned to normal growth media under adherent conditions ( Fig. 2d ). However, when we sorted green-only (miR-200 high) cells and plated them under adherent conditions, within 1 week a substantial number of cells converted to red/green consistent with the reported plasticity of breast cancer non-CSCs to give rise to CSCs [25] . This process was accelerated when cells were cultured under sphere-forming conditions ( Fig. 2e ). These data validated the use of the miR-200 sensors as surrogate markers for CSCs in our experiments, and also confirmed the reported plasticity of CSCs. We have, therefore, used this novel sensor system to explore the effects of stimulation and loss of CD95/CD95L in the context of spontaneous CSCs emergence. MCF-7 cells were infected with the DsRed wt GFP mut sensor and sorted for green cells only, and cultured in the presence of anti-APO-1, LzCD95L or control IgG. Stimulation of CD95 greatly accelerated the appearance of miR-200 low expressing CSCs ( Fig. 2f ); this result was also confirmed in T47D cells ( Fig. 2g ). To determine whether CD95 stimulation regulates the plasticity of CSCs not only by accelerating their spontaneous emergence but also through stabilization of an existing CSC population, we separated the 15% MCF-7 cells with the highest CD24 expression (more differentiated) from the 15% cells with the lowest CD24 expression (less differentiated; Fig. 2h ). After 1 week of culture, we found that the CD24+ cells were unable to repopulate the CD24− cells unless stimulated through CD95. In contrast, the majority of the CD24− cells reverted into the CD24+ population and this was greatly attenuated upon CD95 stimulation. In addition, CD95-mediated apoptosis did not play a role in this process because the effects of CD95 stimulation in both populations could not be inhibited by treatment with zVAD-fmk, which completely blocked CD95-mediated apoptosis (see Supplementary Fig. 2a ). These data suggest that CD95 signalling promotes and maintains the CSC phenotype at least in breast cancer cells. Higher sensitivity of non-CSCs to CD95-mediated apoptosis We previously reported that increasing the concentration of miR-200c in cancer cells increased their sensitivity to CD95-mediated apoptosis [35] . As it is known that overexpression of miR-200c can reduce the stemness of cancer cells [17] , we asked whether CSCs and non-CSCs had differential sensitivities to canonical CD95-mediated apoptosis. To test this, we chose HeyA8 cells, which are highly sensitive to CD95-mediated apoptosis ( Fig. 3a,b ; ref. 9 ). Strikingly, tumour spheres from HeyA8 that showed an increase in ALDH1 activity ( Fig. 3c ) were found to be almost completely resistant to apoptosis induced by CD95 stimulation ( Fig. 3b ). This result was not because of the downregulation of CD95 in the spheres ( Fig. 3d ). Similar results were observed using MCF-7 cells (moderately CD95 apoptosis-sensitive) when plated under sphere-forming conditions ( Fig. 3e ). These data indicate that CSCs are less sensitive to canonical apoptosis induced through CD95 than non-CSCs. 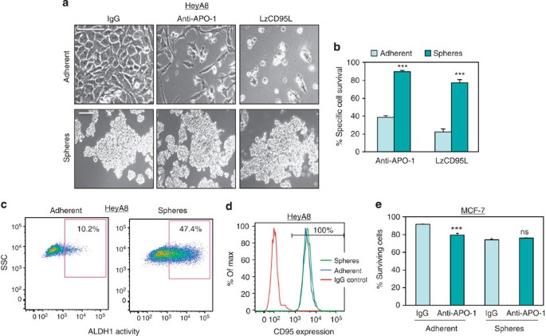Figure 3: CSCs are less sensitive to CD95-mediated apoptosis than non-CSCs. (a)Left:representative images of HeyA8 cells grown for 3 days in the presence of IgG control, anti-APO-1 or LzCD95L under adherence or sphere-forming conditions. Scale bar represents 100 μm. (b) Quantification of surviving cells treated as ina, normalized to IgG controls. Dead cells were quantified using FACS (FSC/SSC gating). Histograms represent mean+s.d. Two independent experiments were performed. (c) ALDH1 activity in HeyA8 cells grown under adherence or sphere-forming conditions. Gates are based on samples co-treated with DEAB-inactivating reagent. (d) CD95 surface expression of HeyA8 cells grown under adherence or sphere-forming conditions. (e) Quantification of surviving MCF-7 cells grown for 6 days in the presence of IgG control or anti-APO-1 under adherence or sphere-forming conditions. Dead cells were quantified with FACS (FSC/SSC gating). Histograms represent mean+s.d. of three independent cultures.Pvalues were calculated byt-test. ***P<0.0001; ns=not significant. Figure 3: CSCs are less sensitive to CD95-mediated apoptosis than non-CSCs. ( a ) Left: representative images of HeyA8 cells grown for 3 days in the presence of IgG control, anti-APO-1 or LzCD95L under adherence or sphere-forming conditions. Scale bar represents 100 μm. ( b ) Quantification of surviving cells treated as in a , normalized to IgG controls. Dead cells were quantified using FACS (FSC/SSC gating). Histograms represent mean+s.d. Two independent experiments were performed. ( c ) ALDH1 activity in HeyA8 cells grown under adherence or sphere-forming conditions. Gates are based on samples co-treated with DEAB-inactivating reagent. ( d ) CD95 surface expression of HeyA8 cells grown under adherence or sphere-forming conditions. ( e ) Quantification of surviving MCF-7 cells grown for 6 days in the presence of IgG control or anti-APO-1 under adherence or sphere-forming conditions. Dead cells were quantified with FACS (FSC/SSC gating). Histograms represent mean+s.d. of three independent cultures. P values were calculated by t -test. *** P <0.0001; ns=not significant. Full size image Elimination of CSCs by induction of DICE The two CT26L clones that formed more spheres than parental CT26 cells (see Fig. 1a ) quantitatively died when DICE was induced [12] , suggesting that CSCs may have an increased sensitivity to DICE. To test this we induced DICE in both MCF-7 and T47D cells by expressing either a CD95- or CD95L-specific short hairpin RNA (shRNA) previously shown to induce DICE ( Fig. 4a,b ). In both cases, cells after DICE initiation lost the population of CD44 high /CD24 low cells suggesting that CSCs could be selectively targeted by DICE. Indeed MCF-7, T47D and HeyA8 cells cultured under sphere-forming conditions were more sensitive to DICE than cells grown under adherent conditions ( Fig. 4c–e ). In addition, after elimination of DICE-sensitive cells using a Tet-inducible shRNA against CD95L [12] the remaining viable HeyA8 cells were less able to form spheres ( Fig. 4f ). Finally, enrichment of CSCs using the miR-200 miRNA sensor also demonstrated increased DICE sensitivity of the flow-sorted miR-200 low expressing MCF-7 cells 7 and 10 days after infection with the pLKO-L3 virus ( Fig. 4g ). 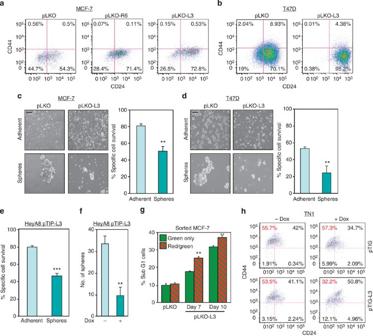Figure 4: CSCs are more sensitive to DICE than non-CSCs. (a,b) Flow cytometry analysis of surface staining of MCF-7 (a) or T47D (b) cells for CD24 and CD44, 9 days after infection with control (pLKO) or with a virus overexpressing shRNAs that targeted CD95 (R6; pLKO-R6) or CD95L (L3; pLKO-L3). Gates are based on isotype controls. Three independent experiments were performed. (c,d)Left:representative images of MCF-7 (c) and T47D (d) cells infected with pLKO or pLKO-L3 viruses seeded under adherence or under sphere-forming conditions and grown for 10 days. Scale bar represents 100 μm.Right:quantification of surviving cells 4 days after plating, assessed with FACS live/dead gating (FSC/SSC). Data for each condition are normalized to pLKO controls. (e) Percent HeyA8-pTIP-L3 cells surviving 5 days after Dox addition, assessed with flow cytometry live/dead gating, normalized to pTIP controls and to Dox-free controls. Histograms represent mean+s.d. of three independent cultures. (f) Numbers of spheres of HeyA8p-pTIP-L3 cells treated with Dox as ine. Histograms represent mean+s.d. of three independent cultures. (g) Percent of flow cytometry-sorted DsRedwtGFPmutgreen or red/green MCF-7 cells in the subG1 fraction (nuclear PI staining) at the indicated times after infection with the pLKO or the pLKO-L3 viruses. Histograms represent mean+s.d. of three independent cultures. (h) CD24/CD44 surface staining of TN1 primary breast cancer cells infected with the pTIG and pTIG-L3 viruses 7 days after Dox addition. Gates are based on isotype controls. Two independent experiments were performed.Pvalues were calculated by ANOVA. **P<0.001; ***P<0.0001. Figure 4: CSCs are more sensitive to DICE than non-CSCs. ( a,b ) Flow cytometry analysis of surface staining of MCF-7 ( a ) or T47D ( b ) cells for CD24 and CD44, 9 days after infection with control (pLKO) or with a virus overexpressing shRNAs that targeted CD95 (R6; pLKO-R6) or CD95L (L3; pLKO-L3). Gates are based on isotype controls. Three independent experiments were performed. ( c , d ) Left: representative images of MCF-7 ( c ) and T47D ( d ) cells infected with pLKO or pLKO-L3 viruses seeded under adherence or under sphere-forming conditions and grown for 10 days. Scale bar represents 100 μm. Right: quantification of surviving cells 4 days after plating, assessed with FACS live/dead gating (FSC/SSC). Data for each condition are normalized to pLKO controls. ( e ) Percent HeyA8-pTIP-L3 cells surviving 5 days after Dox addition, assessed with flow cytometry live/dead gating, normalized to pTIP controls and to Dox-free controls. Histograms represent mean+s.d. of three independent cultures. ( f ) Numbers of spheres of HeyA8p-pTIP-L3 cells treated with Dox as in e . Histograms represent mean+s.d. of three independent cultures. ( g ) Percent of flow cytometry-sorted DsRed wt GFP mut green or red/green MCF-7 cells in the subG1 fraction (nuclear PI staining) at the indicated times after infection with the pLKO or the pLKO-L3 viruses. Histograms represent mean+s.d. of three independent cultures. ( h ) CD24/CD44 surface staining of TN1 primary breast cancer cells infected with the pTIG and pTIG-L3 viruses 7 days after Dox addition. Gates are based on isotype controls. Two independent experiments were performed. P values were calculated by ANOVA. ** P <0.001; *** P <0.0001. Full size image We also tested whether DICE induction would affect CSCs in cancer cell lines of nonbreast or ovarian origin. We tested the colon carcinoma cell line HCT116, the hepatocellular carcinoma cells line HepG2 and the glioblastoma cell line T98G. To achieve a rapid and effective knockdown of CD95 and CD95L, we again expressed the shRNAs targeting either CD95 or CD95L using the Tet-inducible lentiviral vector pTIP [12] . HCT116 cells formed spheres with increased stemness as documented by an increase in CD133 surface expression and ALDH1 activity ( Supplementary Fig. 6a ). After addition of the tetracycline analogue doxycycline (Dox) to HCT116-pTIP-R6 cells (knocking down CD95), the surviving cells showed a reduced ability to form spheres as evidenced by the reduced number and size of HCT116 spheres ( Supplementary Fig. 6b ). To directly test whether CSCs enriched in spheres are more sensitive to DICE, we cultured HCT116-pTIP control cells and HCT116-pTIP-R6 cells under sphere-forming conditions resulting in the formation of spherical structures. Five days after addition of Dox, pTIP control-expressing cells maintained their sphere-forming ability. In contrast, HCT116-pTIP-R6 cells failed to form spheres but assumed rather unstructured clumps of cells and exhibited a decrease in cell viability ( Supplementary Fig. 6c ). Surface staining for CD133 and ALDH1 activity confirmed that DICE induction caused a reduction of CSCs ( Supplementary Fig. 6d ), and a cell death assay showed reduced viability of these cells as well as of HepG2-pTIP-L3 and T98G-pTIP-L3 cells when grown under sphere-forming conditions ( Supplementary Fig. 6e ). To determine whether primary CSCs isolated from a patient also showed increased susceptibility to DICE, we isolated cells from a patient-derived human-in-mouse xenografted model (PDX) of a primary triple-negative breast cancer (TN1) containing a high percentage of CD44 high CD24 low CSCs [36] . These cells were isolated from mice, briefly infected with a GFP-expressing version of the inducible shL3 (pTIG-L3 (ref. 12 )) and plated in the presence of Dox ( Fig. 4h ). Similar to the results obtained with breast cancer cell lines, these PDX mouse-derived human cells (and only when expressing pTIG-L3) showed a clear reduction in CD44 high cells 7 days after Dox addition, suggesting that the CSCs in general have an increased sensitivity to DICE. Finally, to determine whether a knockout (as opposed to knockdown) of CD95 would also result in elimination of CSCs, we used a mouse ovarian cancer cell line we recently described to express oncogenic Kras and carrying a deletion of both alleles of Pten but with both alleles of CD95 flanked by loxP sites (clone no. 6 in ref. 12 ). When infected with Adenoviral (AdV) GFP-Cre, which resulted in the deletion of both CD95 alleles ( Supplementary Fig. 7a ), cells showed signs of distress and slowed down in growth ( Supplementary Fig. 7b ). However, as high Cre expression can be toxic to cells [37] it was not clear whether this was caused by ongoing DICE. In order to eliminate any traces of AdV genes and to be certain that cells did not contain any unrecombined CD95, we cultured the cells for 7 weeks and then performed single cell cloning. We picked three clones of the cells treated with AdV-GFP control virus and three of the cells infected with AdV-GFP-Cre and found no traces of WT CD95 in the Cre-treated cells using PCR ( Supplementary Fig. 7c ) or western blot analysis ( Supplementary Fig. 7d ). Interestingly, we detected an 80% reduction in CSCs in the CD95-deficient cells ( Supplementary Fig. 7e ), confirming the results obtained with shRNAs, that CD95 promotes the survival of CSCs. Modulating sensitivity to CD95-mediated apoptosis and to DICE In breast cancer, miR-200 expression is characteristic for non-CSCs and miR-221 expression is enriched in CSCs [38] . MCF-7 cells are miR-200 high/miR-221 low (CD44 low CD24 high ) expressing cells with an epithelial character, contain low numbers of CSCs and exhibit moderate sensitivity to CD95-mediated apoptosis. In contrast, highly metastatic MDA-MB-231 cells are miR-200 low/miR-221 high expressing cells, are almost exclusively CD44 high CD24 low mesenchymal cells and are completely resistant to CD95-mediated apoptosis ( Supplementary Fig. 8a–e ). Consistent with our data that cells with CSC properties are more sensitive to DICE than non-CSCs, MDA-MB-231 cells were more susceptible to DICE than MCF-7 cells ( Supplementary Fig. 8b ). To test whether the number of CSCs could be changed along with the sensitivity to DICE by altering miR-200 expression levels in cancer cells, we stably overexpressed miR-200c in MDA-MB-231 cells ( Fig. 5a , Supplementary Fig. 12 ). This resulted in decreased expression of the CSC-associated miR-221 ( Fig. 5a ), the miR-200 targets and SC factors BMI1, SOX2, and ZEB1 (ref. 39 ) and by a reduced ability of the cells to form spheres ( Fig. 5b ). When DICE was induced by knocking down CD95L ( Fig. 5c ), which results in upregulation of miR-200b/c and downregulation of miR-221 ( Fig. 5d ), miR-200c-overexpressing cells showed significantly reduced sensitivity, consistent with our observation that DICE preferentially kills CSCs ( Fig. 5e ). 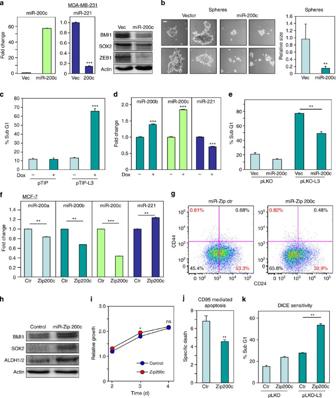Figure 5: Modulating sensitivity to CD95-mediated apoptosis and to DICE. (a)Left:real-time PCR quantification of miR-200c and miR-221 expression in MDA-MB-231 stably expressing pre-miR-200c compared with control vector-infected cells. Data are normalized to vector-infected cells. Histograms represent mean+s.d. of three independent measurements.Right:western blot analysis of the same cells. (b) Representative images and sphere area quantification of vector and pre-miR-200c-infected MDA-MB-231 cells after a 1-week culture under sphere-forming conditions. Scale bar represents 100 μm. Area quantification was carried out using Image-J.Pvalues were calculated byt-test. Histograms represent mean+s.d. of measurements from three independent cultures. (c) Percent cell death (nuclear PI staining) 5 days after Dox addition of MDA-MB-231-pTIP and pTIP-L3 cells.Pvalues were calculated by ANOVA. Histograms represent mean+s.d. of three independent cultures. Two independent experiments were performed. (d) Real-time PCR quantification of miR-200b, miR-200c and miR-221 in MDA-MB-231-pTIP-L3 cells 6 days after Dox addition, normalized to pTIP controls.Pvalues were calculated by ANOVA. Histograms represent mean+s.d. of three independent measurements. (e) Percent cell death (nuclear PI staining) of vector control and miR-200c overexpressing MDA-MB-231 cells 7 days after infection with pLKO or pLKO-L3.Pvalues were calculated by ANOVA. Histograms represent mean+s.d. of three independent cultures. Two independent experiments were performed. (f) miR-200a, miR-200b, miR-200c and miR-221 expression levels in MCF-7 infected with vector control or with the Zip200c virus. Histograms represent mean+s.d. of three independent measurements. (g) CD24 and CD44 surface staining of MCF-7 cells infected with control or Zip200c virus. Gates are based on isotype controls. Three independent experiments were performed. (h) Western blot analysis of MCF-7 cells infected with control or Zip200c virus, with actin as a loading control. (i) MTS proliferation assay of MCF-7 cells infected with vector or with Zip200c, normalized to day 1.Pvalues were calculated byt-test. Data represent mean±s.d. of four independent cultures. (j,k). Effects of CD95 stimulation (j) and CD95L knockdown (k) on viability of MCF-7 cells infected with control or Zip200c virus. Specific death was assessed as percent subG1 cells (nuclear PI staining), normalized to IgG-treated controls. Histograms represent mean+s.d. of three independent cultures.Pvalues were calculated by ANOVA. *P<0.05; **P<0.001; ***P<0.0001. Figure 5: Modulating sensitivity to CD95-mediated apoptosis and to DICE. ( a ) Left: real-time PCR quantification of miR-200c and miR-221 expression in MDA-MB-231 stably expressing pre-miR-200c compared with control vector-infected cells. Data are normalized to vector-infected cells. Histograms represent mean+s.d. of three independent measurements. Right: western blot analysis of the same cells. ( b ) Representative images and sphere area quantification of vector and pre-miR-200c-infected MDA-MB-231 cells after a 1-week culture under sphere-forming conditions. Scale bar represents 100 μm. Area quantification was carried out using Image-J. P values were calculated by t -test. Histograms represent mean+s.d. of measurements from three independent cultures. ( c ) Percent cell death (nuclear PI staining) 5 days after Dox addition of MDA-MB-231-pTIP and pTIP-L3 cells. P values were calculated by ANOVA. Histograms represent mean+s.d. of three independent cultures. Two independent experiments were performed. ( d ) Real-time PCR quantification of miR-200b, miR-200c and miR-221 in MDA-MB-231-pTIP-L3 cells 6 days after Dox addition, normalized to pTIP controls. P values were calculated by ANOVA. Histograms represent mean+s.d. of three independent measurements. ( e ) Percent cell death (nuclear PI staining) of vector control and miR-200c overexpressing MDA-MB-231 cells 7 days after infection with pLKO or pLKO-L3. P values were calculated by ANOVA. Histograms represent mean+s.d. of three independent cultures. Two independent experiments were performed. ( f ) miR-200a, miR-200b, miR-200c and miR-221 expression levels in MCF-7 infected with vector control or with the Zip200c virus. Histograms represent mean+s.d. of three independent measurements. ( g ) CD24 and CD44 surface staining of MCF-7 cells infected with control or Zip200c virus. Gates are based on isotype controls. Three independent experiments were performed. ( h ) Western blot analysis of MCF-7 cells infected with control or Zip200c virus, with actin as a loading control. ( i ) MTS proliferation assay of MCF-7 cells infected with vector or with Zip200c, normalized to day 1. P values were calculated by t -test. Data represent mean±s.d. of four independent cultures. ( j , k ). Effects of CD95 stimulation ( j ) and CD95L knockdown ( k ) on viability of MCF-7 cells infected with control or Zip200c virus. Specific death was assessed as percent subG1 cells (nuclear PI staining), normalized to IgG-treated controls. Histograms represent mean+s.d. of three independent cultures. P values were calculated by ANOVA. * P <0.05; ** P <0.001; *** P <0.0001. Full size image Finally, to test whether inhibition of miR-200 expression would increase stemness of breast cancer cells resulting in increased sensitivity to DICE, we infected MCF-7 cells with a lentiviral inhibitor of miR-200c (Zip200c; Fig. 5f ). This caused a slight increase in the fraction of CD44 high cells, a significant decrease in the CD24 high population ( Fig. 5g ) and an increase in expression of the CSC markers miR-221 ( Fig. 5f ), BMI1, SOX2 and ALDH1/2 ( Fig. 5h ). No significant difference in the growth rate between control and miR-200 knockdown cells was detected ( Fig. 5i ). These cells induced to have increased CSC content showed reduced sensitivity to CD95-mediated apoptosis ( Fig. 5j ) and a significant increase in sensitivity to DICE ( Fig. 5k ). These results indicate that miR-200 is not only a negative marker for breast CSCs, but is functionally connected to the role of CD95, specifically in CSCs and determines the sensitivity of cancer cells to DICE. Synergism between DICE- and CD95-mediated apoptosis Our data demonstrate that stimulation of CD95 on cancer cells or reducing miR-200c levels increases the number of CSCs, which are more sensitive to induction of DICE than non-CSCs, but less sensitive to CD95-mediated apoptosis. In contrast, induction of DICE or overexpression of miR-200c reduces the number of CSCs, increasing the number of non-CSCs, which are more sensitive to CD95-mediated apoptosis. This suggested that the concomitant induction of DICE and of CD95-mediated apoptosis may kill both CSCs and non-CSCs. To test this hypothesis, we knocked down either CD95 or CD95L in MCF-7 cells by infecting them with pLKO lentiviruses expressing either the R6 or L3 shRNAs, and 6 days after infection cells were treated with anti-APO-1 for an additional 4 days. At this time point, MCF-7 cells infected with a control virus were moderately sensitive to CD95-induced apoptosis ( Fig. 6a ). Knockdown of CD95, while inducing DICE in ~15% of the cells, did not significantly alter the apoptosis sensitivity of the cells. This was not surprising considering that CD95 expression was significantly reduced (inset in Fig. 6a ). In contrast, when CD95L was knocked down, it caused DICE induction in ~21% of the cells and the concomitant stimulation of CD95 with anti-APO-1 substantially increased cell death to almost 90% ( Fig. 6a ). Part of the increase in apoptosis induction could be explained by a slight increase in surface expression of CD95 after knockdown of CD95L ( Fig. 6a ). Similar findings were made with HeyA8 cells; however, because of the high CD95 apoptosis sensitivity of these cells, shorter kinetics were used to induce apoptosis or DICE ( Fig. 6b ). These results are consistent with the elimination of CSCs by DICE, followed by efficient apoptosis induction in the remaining DICE-resistant non-CSCs. These data suggest that cancer cells consist of non-CSCs that can be sensitive to canonical CD95-mediated apoptosis and a CSC population, which can be targeted by DICE. 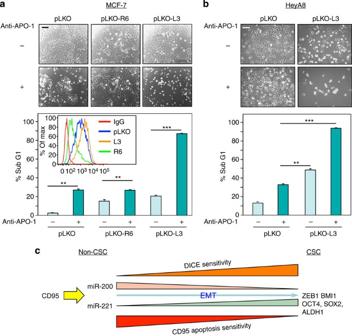Figure 6: Synergism between DICE and CD95-mediated apoptosis. Effects of DICE achieved by infection with pLKO-R6 or pLKO-L3 in combination with anti-APO-1 in (a) MCF-7 cells 9 days after infection and (b) HeyA8 cells 6 days after infection (including 2 days of puromycin selection). Anti-APO-1 was added to the cell culture during the last 4 and 3 days, respectively. Scale bar represents 100 μm. Death was assayed with FACS analysis by nuclear PI staining. Histograms represent mean+s.d. of three independent cultures. Two independent experiments were performed. Inset inashows surface expression of CD95 in MCF-7 cells 10 days after infection with pLKO, R6 or L3 virus. Isotype-matched IgG was used as control. Two independent experiments were performed.Pvalues were calculated by ANOVA. **P<0.001; ***P<0.0001. (c) Scheme illustrating the activity of CD95 to maintain CSCs. CD95 stimulation is driving both EMT and emergence of CSCs. This results in the loss of miR-200 expression upregulation of stem cell regulating transcription factors (and in breast cancer, increased expression of miR-221). While undergoing EMT and developing CSC traits, cells gradually lose sensitivity to CD95-mediated apoptosis and become more and more dependent on the expression of both CD95 and CD95L. When either of these molecules are removed from cancer cells, they undergo DICE. Figure 6: Synergism between DICE and CD95-mediated apoptosis. Effects of DICE achieved by infection with pLKO-R6 or pLKO-L3 in combination with anti-APO-1 in ( a ) MCF-7 cells 9 days after infection and ( b ) HeyA8 cells 6 days after infection (including 2 days of puromycin selection). Anti-APO-1 was added to the cell culture during the last 4 and 3 days, respectively. Scale bar represents 100 μm. Death was assayed with FACS analysis by nuclear PI staining. Histograms represent mean+s.d. of three independent cultures. Two independent experiments were performed. Inset in a shows surface expression of CD95 in MCF-7 cells 10 days after infection with pLKO, R6 or L3 virus. Isotype-matched IgG was used as control. Two independent experiments were performed. P values were calculated by ANOVA. ** P <0.001; *** P <0.0001. ( c ) Scheme illustrating the activity of CD95 to maintain CSCs. CD95 stimulation is driving both EMT and emergence of CSCs. This results in the loss of miR-200 expression upregulation of stem cell regulating transcription factors (and in breast cancer, increased expression of miR-221). While undergoing EMT and developing CSC traits, cells gradually lose sensitivity to CD95-mediated apoptosis and become more and more dependent on the expression of both CD95 and CD95L. When either of these molecules are removed from cancer cells, they undergo DICE. Full size image We recently reported that DICE could be induced in all of the 12 tested cancer cell lines [12] but that the percentage of cells that died through DICE varied across different cell lines. We now provide evidence that DICE predominantly affects CSCs, and that DICE can be more efficiently induced in cancer cell populations with a higher CSC content. In contrast, induction of canonical CD95-mediated apoptosis preferentially targets non-CSCs. Consequently, either enriching cancer cells for CSCs (by sorting through surface markers or miR-200 expression, or growth under sphere-forming conditions) or converting them (by altering miR-200 levels or stimulation through CD95) resulted in a reciprocal change in sensitivity to DICE or to CD95-mediated apoptosis ( Fig. 6c ). In addition to our findings on the differential sensitivity of different cancer cell populations to DICE- and CD95-mediated apoptosis, we have uncovered a new function of CD95. CD95 expression is beneficial to cancer cells because it can transform cancer cells into a more de-differentiated state. Our findings suggest that in addition to eliminating differentiated cells through induction of apoptosis (which happens quickly) CD95 converts apoptosis-resistant differentiated cells, or non-CSCs, into CSCs (this can take many days) and maintains CSCs. The data are consistent with recent reports that described CD95 as a driver of the EMT in cancer cells [40] , [41] . Interestingly, in breast cancer, a clear connection between EMT and the formation of CSCs has been established [16] , [17] . A number of earlier publications demonstrated that when cancer cells (or tissue grafts) were engineered to express exogenous CD95L and grown in vivo they were rejected more rapidly than cells expressing a control vector due to neutrophilic destruction of the graft [42] , [43] . Surprisingly, HeyA8 expressing CD95L used in our study were not rejected when injected into NSG mice. NSG mice have never been used before for these kind of studies but neutrophilic granulocytes are present in these mice [44] . Our data suggest that neutrophils are not destroying CD95L-expressing cancer cells under all circumstances. While we mostly concentrated on breast cancer, because of their well-described CSC properties, in terms of surface markers (CD24 and CD44) [20] , [31] , our data are likely not limited to breast cancer. We made similar observations in cancer cells of other tissue origin including the ovary, colon, liver and brain, suggesting that the activities of CD95 we describe could be of general importance to cancer. Inspired by previous reports [45] , [46] , we have generated a fluorescence-based lentiviral sensor system that allowed us to monitor the expression of miR-200 in living cells. In contrast to most CSC markers, miR-200c has a well-described activity as a regulator of stemness of cancer cells [19] . In contrast to previous constructs, which relied on seed sequences with complete complementarity to the detected miRNA, we chose a piece of the 3′-UTR of a natural substrate, ZEB2, as a miR-200 sensor. This sensor system was able to enrich and allowed to isolate cancer cells with CSC features, and could detect an increase in the CSC population in breast cancer cells upon CD95 stimulation. Conversely, CSCs isolated through the activity of miR-200 were significantly more sensitive to CD95 knockdown than non-CSCs. These data are complementary to our previous report in which we demonstrated that overexpression of miR-200 rendered cancer cells more susceptible to CD95-mediated apoptosis [35] . Our data on multiple cancer cell lines and primary triple-negative breast cancer cells passaged in PDX mice demonstrate that DICE predominantly affects CSCs, suggesting that it might be possible to deplete cancer of CSCs by inducing DICE. We recently proposed a model in which we discussed DICE as an yet unidentified cancer surveillance mechanism [13] . According to this model, neoplastically transformed cells undergo DICE when they acquire mutations that render CD95 inactive as this would prevent immune cells from killing cancer cells through CD95. Furthermore, because CD95L is produced by cancer cells to provide low level survival signalling through CD95 mutations in the CD95L gene would have the same effect. The fact that among cancer cells, CSCs are most sensitive to DICE induction may be a reflection of the fact that SCs need to be especially protected from undergoing neoplastic transformation. We suggest that inducing stemness will increase the susceptibility of cancer cells to DICE. One might argue that increasing stemness of cancer cells (for example, by inhibiting miR-200) may result in increased numbers of therapy-resistant and metastatic cells, which would be deleterious. However, the clinical reality needs to be considered. Most patients die from treatment-refractory and highly metastatic diseases. It has been shown multiple times that cancer in such patients contains an increased number of CSCs [31] , [47] . Thus, there is likely no need to deliberately increase the number of CSCs in patients because that may have already been caused by the conventional treatment. Our data suggest that induction of DICE combined with induction of canonical CD95-mediated apoptosis should result in an almost complete elimination of cancer cells. While treating cancer patients systemically with CD95L will not be possible because of its toxicity, our data suggest that the elimination of DICE-sensitive cancer cells should result in cells with reduced stemness and most importantly increased sensitivity to CD95-mediated apoptosis, perhaps giving the immune system an opportunity to eliminate these remaining cancer cells. Cell Lines The breast cancer cell lines MCF-7, T47D and MDA-MB-231, the renal carcinoma cell line CAKI-1 (obtained from the ATCC) and the ovarian cancer cell line HeyA8 (obtained from Dr E. Lengyel, University of Chicago) were cultured in RPMI-1640 medium (Mediatech Inc) containing 10% heat-inactivated fetal bovine serum (FBS; Sigma-Aldrich) and 1% penicillin/streptomycin (Mediatech Inc). The hepatocellular carcinoma cell line HepG2 (ATCC) was cultured in EMEM (ATCC) and the glioblastoma cell line T98G in DMEM (Mediatech Inc). The colon carcinoma cell line HCT116 (ATCC) was cultured in McCoy’s 5A medium (ATCC). CT26 cells (ATCC) and CT26L cells obtained from Dr G. Nabel [48] , which express human CD95L, were cultured in DMEM medium (Mediatech Inc) containing 10% heat-inactivated FBS and 1% penicillin/streptomycin. CT26-pTIP-L3 clones no. 18 and no. 22 were recently generated [12] . All other cell lines stably expressing shRNAs and Tet-inducible shRNAs targeting either CD95 or CD95L (using either pTIP or pTIG vectors) were described recently [12] . MDA-MB-231 cells expressing control (pLNCX2) and pre-miR-200c were maintained in RPMI with 1 μg ml −1 G418 (Sigma). MCF-7 cells overexpressing miR-Zip anti-miRNA control and anti-miR-200c (System Biosciences) were maintained in RPMI with 3 μg ml −1 puromycin. MCF-7-vec and MCF-7-CD95L and HeyA8-vec and HeyA8-CD95L cells were generated by infecting MCF-7 and HeyA8 cells with pLenti-GIII-CMV-RFP-Puro or pLenti-GIII-CMV-RFP-2A-Puro-CD95L (accession number BC017502, ABM) and selected with 3 μg ml −1 puromycin. Proteins resulting from infection with the third-generation lentiviruses from ABM carry some additional amino acids at the C terminus. We confirmed that the CD95L used was active in inducing CD95-mediated apoptosis when expressed in HeyA8 cells ( Supplementary Fig. 9 ). Reagents and antibodies Reagents used for western blot analysis were obtained from the following sources (all primary antibodies were used at a 1:1,000 dilution, unless otherwise specified): Anti-ß-actin antibody (Clone no. I-19; 1:500), anti-hCD95 sc-715 (C-20), anti-mCD95 sc-1024 (X-20), anti-hCD24 (ALB9), anti-hCD44 (HCAM BU52), BMI-1 (F-9) and ALDH1/2 (H-85) were from Santa Cruz Biotechnology, USA. Anti-hSOX2 and anti-hOCT4 were from Cell Signaling. Anti-ZEB1 (HPA027524) was from Sigma. Anti-hE-Cadherin no. 205601 was from Calbiochem. Anti-hCD95L (no. 556387; 1:500) was from BD Biosciences. All secondary antibodies were used at a 1:5,000 dilution: goat anti-rat IgG, HRP-conjugated (Enzo Life Science); goat anti-mouse IgG, horseradish peroxidase-conjugated, rabbit anti-goat IgG, HRP-conjugated and goat anti-rabbit IgG, HRP-conjugated (Southern Biotech). Reagents used for flow cytometry, CD24-APC (0.025 μg per sample), CD44-PE-Cy7 (0.06 μg per sample) and isotype controls were from eBioscience, CD133 (AC133, 1:10 dilution) and isotype control antibody from Miltenyi Biotech. The Aldefluor kit (Stem Cell Technologies) was used for the staining and quantification of ALDH1 activity with flow cytometry. Gates were based on the analysis of cells treated with the specific inhibiting reagent DEAB as a negative control following the instructions by the manufacturer. CD95 surface staining was performed with the anti-APO-1 antibody [49] (1 μg ml −1 ). Primary breast cancer cells, TN1, were stained with anti-mouse H2K-biotin, streptavidin-PE-Cy7, CD44-APC (0.025 μg per sample) and CD24-PE (0.025 μg per sample) from BD. Bovine serum albumin (BSA), Dox, puromycin, G418, protein A, propidium iodide were from Sigma and 4',6-diamidino-2-phenylindole (DAPI) was from VECTOR Laboratories Inc. CFSE and 7AAD were from Life Technologies. zVAD-fmk caspase inhibitor (used at 20 μM) was from Santa Cruz Biotechnology. Anti-CD95 mAb anti-APO-1 and leucine zipper-tagged CD95L (LzCD95L) were used to induce apoptosis at 100 ng ml −1 . In all cases when anti-APO-1 or control IgG was used to stimulate cells, 1 ng ml −1 of Protein A (Sigma) was added to crosslink the antibodies. Knockdown using lentiviral shRNAs Cells were infected with the following MISSION Lentiviral Transduction Particles (Sigma): pLKO.2-puro Control Transduction Particle coding for a nontargeting (scrambled) shRNA, pLKO (no. SHC002; CCGGCAACAAGATG AAGAGCACCAACTCGAGTTGGTGCTCTTCATCTTGTTGTTTTT), shRNA against mRNA NM_000639 (Homo sapiens Fas ligand, shFASL), TRCN0000059000 (L3: CCGGACTGGGCTGTACTTTGTATATCTCGAGATATACAAAGTACAGCCCAGTTTTTTG, and shRNA against mRNA NM_000043 (Homo sapiens Fas) TRCN0000038696 (R6: CCGGGTGCAG ATGTAAACCAAACTTCTCGA GAAGTTTGGTTTACATCTGCACTTTTTG). In all, 50,000 cells seeded in six-well plates were infected with each lentivirus at a multiplicity of infection of 3 in the presence of 8 μg ml −1 polybrene. Cells were cultured in selection medium containing 3 μg ml −1 of puromycin for 2 days. In all experiments involving puromycin selection, mock-infected cells were included and were also treated with puromycin. Cells were only analysed after all such non-infected cells died within 2–3 days after addition of puromycin. Western blot analysis Cells were lysed in RIPA lysis buffer (1% SDS, 1% Triton X-100, 1% deoxycholic acid) and quantified using the DC Protein Assay kit (Bio-Rad). Proteins (25–50 μg) in lysates were resolved on 12% SDS–PAGE gels and transferred to nitrocellulose membrane (Protran, Whatman). The membranes were blocked with 5% non-fat dry milk in 0.1% TBS/Tween-20 or 2% BSA-TBS/Tween-20 (CD95, CD95L and E-cadherin) and incubated in primary antibodies diluted in blocking solution at 4 °C overnight. After incubation with secondary antibodies, detection was performed using the ECL method (Amersham Pharmacia Biotech) and developed using a chemiluminescence imager, G:BOX Chemi XT4 (Synoptics). The uncropped scanned films with molecular weight reference are included in Supplementary Fig. 10 through 12 in sequence of appearance in the main text. Immunofluorescence and FACS analysis Cells were washed twice in PBS with 2% BSA and stained with primary antibody for 45 min at 4 °C in the dark. Cells were then washed and centrifuged twice at 500 g and incubated with secondary antibody for an additional 30 min. After an additional centrifugation, cells were stored on ice until fluorescence-activated cell sorting (FACS) analysis, which was performed on a Becton Dickinson LSR Fortessa. Data were analysed using FlowJo version 8.8.6 (Treestar Inc). DAPI staining and FSC-A and SSC-A gating were used to exclude dead cells and FSC-W, and SSC-W gating was applied to exclude doublets. When needed, cell sorting was performed on a Beckman Coulter MoFlo sorter. Sphere-forming assay Cells (0.1–0.5 × 10 4 ) were collected, washed in PBS and seeded in triplicates on Ultra-Low attachment multiwell plates (Corning) in Mammocult cancer stem cell medium (Cell Stem Technology), prepared according to the manufacturer’s instruction. Seven days after plating, spheres were either passaged and replated (either under adherence or non-adherent conditions), stained or counted using a light microscope. Sphere size was quantified on acquired images using Image J v. 1.44. Images of fluorescently labelled cells were taken and analysed with an Axiovert S100 immunofluorescence microscope equipped with an Axiocam digital camera and software (Zeiss). Generation of cells stably expressing a miR-200 sensor The sensor plasmid was generated by linking fragments of the ZEB2 3′-UTR (from the 782 to 1,080 portion of the ZEB2 3′-UTR, containing miR-200 seed numbers 4, 5 and 6 (ref. 15 )) to GFP (pAcGFP1-Hyg-C1) and DsRed (pDsRed-Express-C1) containing plasmids (from Clontech Laboratories). As inactive controls, mutated versions of the 3′-UTRs were generated (synthesis by IDT Technologies), mutating the miR-200 seed matches from CAGTATT to CTGAAAT to prevent miRNA targeting. GFP-3′-UTR or DsRed-3′-UTR either wt or mutated were cloned in tandem into a CD510B-1 lentivector (from System Biosciences) driven by two identical CMV promoters. The restriction enzymes flanking the 3′-UTRs were NotI and Xho1 on one side and PmlI and SalI on the other side. A scheme of the sensor double-CMV plasmid is shown in Supplementary Fig. 3a . The plasmid was used to generate viruses with pCMVDR8.9 (packaging) and pMD.G (envelope) plasmids in 293T cells and target cells were infected with the filtered supernatant in the presence of 8 μg ml −1 polybrene. Fluorescence was monitored 72 h post infection on a fluorescence microscope or with FACS. Testing the miRNA sensor 293T cells (0.1–0.2 × 10 5 ) were seeded in 12-well plates 1 day before transfection. Cells were transfected with Lipofectamine 2000 (Invitrogen) and with different concentrations of pre-nontargeting control, pre-miR-200a, 200b, 200c, 141 or 429 (Ambion) or an LNA-based panspecific miRNA-200 inhibitor [15] . Seventy-two hours post transfection, cells were harvested, and green and red fluorescence were quantified by FACS analysis. Real-time PCR and quantification of miRNA Total RNA was extracted using the miRNeasy Mini kit (Qiagen) following the manufacturer’s protocol. For miRNA quantitation, 30–60 ng of RNA was reverse-transcribed with the high-capacity cDNA reverse transcription kit (Applied Biosystems), and cDNA was quantitated using primers for miR-200a, miR-200b, miR-200c, miR-221 and RNUB6 (housekeeping control). Results were normalized to RNUB6 (miRNA expression) by the use of the comparative Δ C T method, and expressed as fold differences. Proliferation Assay (MTS) Cells were seeded in 96-well plates and incubated at 37 °C. Cell viability was determined in triplicate at various time points using the MTS assay according to the manufacturer’s instructions (Promega). Plates were analysed at OD 490 using an iMark Microplate Reader (Bio-rad). Data are represented as means±s.d. CFSE staining In all, 500,000 cells were incubated with 10 μM CFSE (Molecular Probes) in PBS for 10 min at 37 °C. Cells were washed with 5 volumes of ice-cold PBS and left on ice for 5 min, then washed three times in warm media and either analysed by FACS or replated. Dead cells were excluded by 7AAD staining, which was carried out by adding 5 μl of a 1-mg ml −1 solution of 7AAD to 200 μl of cells and incubated for 30 min at 4 °C in the dark. Cell death assays Different cell death assays were used, depending on specific experimental requirements. To quantify DNA fragmentation after a treatment, both dead and live cells were collected for the assay. The total cell pellet was resuspended in 0.1% sodium citrate, pH 7.4, 0.05% Triton X-100 and 50 μg ml −1 propidium iodide. After 2–4 h in the dark at 4 °C, fragmented DNA (% subG1 nuclei) was quantified with flow cytometry. To stain cells with DAPI, after a treatment, both dead and live cells were collected and resuspended in 200–300 μl of media, and DAPI was added at 0.025 mg ml −1 . Percent dead cells (DAPI-positive) was monitored using FACS in combination with FSC-A and SSC-A gating. To quantify cell death using the trypan blue exclusion assay, cells were resuspended in media and an equal volume of Trypan blue solution (Cellgro) was added. Both living and dead (blue) cells were counted on a haemocytometer under a light microscope. Injection into NSG mice and in vivo imaging In all, 100,000 HeyA8-pTIG or HeyA8-pTIG-L3 cells also infected with pFU-L2G [36] luciferase lentivirus were injected i.p. into 6-week-old female NSG mice (Jackson lab) according to the Northwestern University Institutional Animal Care and Use Committee (IACUC)-approved protocol. The growth of cells was monitored by using the IVIS Spectrum in vivo imaging system and luminescence was quantified at the regions of interest (the same area for each mouse encompassing the entire abdomen) with the Living Image software. Infection and staining of primary breast cancer cells Primary triple-negative breast cancer cells (TN1) passaged in NOD/severe combined immunodeficiency mice [37] under a protocol approved by the Case Western Reserve University IACUC. Cells were isolated from the tumours after mincing small tumour pieces and digesting with Collagenase III (3,000 units ml −1 in HBSS, Worthington Biomedical) and 100 Kunitz units of DNase I (D4263; Sigma) at 37 °C for 2 h (pipetted six times, once every 20 min). Single cells were isolated using a 40-mm-nylon strainer. RPMI-1640 medium containing 10% FBS was added to inactivate the protease. Cells were spun down and resuspended in HBSS/2% FBS. Cells were infected for 3 h in the presence of polybrene 8 μg ml −1 with either the pTIG or the pTIG-L3 virus (expressing GFP) and then plated on collagen I coated (5 μg per well) 96 wells in HuMEC media (Life Technology) containing 100 ng ml −1 Dox. Cells were collected 7 days after Dox addition and stained with anti-mouse H2K-biotin, streptavidin-PE-Cy7, CD44-APC and CD24-PE. The histograms in Fig. 4h show the CD24/CD44 staining on DAPI-negative/H2K-negative/GFP-positive gated cells. Generation of CD95 KO ovarian cancer cell clones We previously described a cell line isolated from an ovarian cancer that grew in Kras G12D/wt Pten loxP/loxP CD95 loxP/loxP Amhr2 Cre/wt mice [12] . While this cell line had recombined Kras G12D/wt and deleted both alleles of Pten , it still had two intact CD95 loxP alleles (see clone no. 6 in Fig. 7C in (ref. 12 )). In order to generate cancer cells with both alleles of CD95 completely knocked out (exon 9 deletion), cells were infected with GFP-Cre adenovirus (AdV; obtained from the University of Iowa Gene Transfer Vector Core) at 50–100 multiplicity of infection or an AdV-GFP control virus. Three days after infection, cells were observed under the microscope and the status of the CD95 locus was analysed by genotyping. No recombination was observed in the control-infected cells and efficient recombination of CD95 loxP/loxP was seen in cells infected with AdV-GFP-Cre (see Supplementary Fig. 7a ). To be absolutely certain that no CD95-expressing cells would be present in the culture after knockout of CD95, cells were subjected to single cell cloning at one cell per well. Before this step, cells were cultured for 7 weeks to be sure that no AdV was present anymore. Two weeks after single-cell culture, three clones of each (AdV-GFP and AdV-GFP-Cre-treated cells) were randomly selected, genotyped for Pten and CD95 using the following primers: Pten WT forward: ACTCAAGGCAGGGATGAGC; Pten WT (left loxP) reverse: AATCTAGGGCCTCTTGTGCC; Pten KO forward: ACTCAAGGCAGGGATGAGC; Pten KO reverse: GCTTGATATCGAATTCCTGCAGC; CD95 right loxP forward: GCTGTGTCTATCAGTCTC; CD95 right loxP reverse: AAGAGACCCACCTCTAGGTAG; CD95 WT (exon 9) forward: ATGCATGACAGCATCCAAGA; CD95 WT (exon 9) reverse: TGCTGGCAAAGAGAACACAC; CD95 KO forward: CTGTGGTGGGAGAACTGGAT; CD95 KO reverse: TGGGTATGCTCCAGATAGGC. Cells were subjected to western blot analysis for the expression of muCD95 and analysed for the activity of the CSC marker ALDH1 using the Aldefluor assay and flow cytometry. Statistical analysis All experiments were performed in triplicate. The results were expressed as mean±s.d. and analysed by the Student’s two-tailed t -test or by analysis of variance (Statplus v.5.8). Statistical significance was defined as P <0.05. How to cite this article : Ceppi, P. et al. CD95 and CD95L promote and protect cancer stem cells. Nat. Commun. 5:5238 doi: 10.1038/ncomms6238 (2014).